Emergence of non-centrosymmetric topological insulating phase in BiTeI under pressure The spin–orbit interaction affects the electronic structure of solids in various ways. Topological insulators are one example in which the spin–orbit interaction leads the bulk bands to have a non-trivial topology, observable as gapless surface or edge states. Another example is the Rashba effect, which lifts the electron-spin degeneracy as a consequence of the spin–orbit interaction under broken inversion symmetry. It is of particular importance to know how these two effects, that is, the non-trivial topology of electronic states and the Rashba spin splitting, interplay with each other. Here we show through sophisticated first-principles calculations that BiTeI, a giant bulk Rashba semiconductor, turns into a topological insulator under a reasonable pressure. This material is shown to exhibit several unique features, such as a highly pressure-tunable giant Rashba spin splitting, an unusual pressure-induced quantum phase transition, and more importantly, the formation of strikingly different Dirac surface states at opposite sides of the material. The theoretical work of Kane and Mele [1] has marked a milestone in our understanding of the insulating phase of the matter. In their seminal work, they classified the bulk insulators according to the topological order of their electronic states using quantum metrics known as topological indices. When nontrivially ordered, it was predicted that such topological insulators (TIs) should exhibit gapless states at their boundaries, for example, at the surface or edges. The succeeding works have confirmed this prediction by theoretically proposing and/or experimentally discovering a number of two- and three-dimensional TIs, including HgTe quantum wells [2] , [3] and uniaxially strained bulk HgTe [4] , [5] , a number of layered V 2 VI 3 binary compounds, for example, Bi 2 Se 3 , Bi 2 Te 3 , and Sb 2 Te 3 [6] , [7] , and the ternary compounds LaBiTe 3 [8] , TlBiTe 2 and TlBiSe 2 [9] , [10] . The recent first-principles studies have further proposed that several half-Heusler compounds, such as LaPtBi, LuPtSb and YPdBi [11] , [12] , [13] , [14] , can turn into a TI under a uniaxial strain, similar to what was predicted and observed for HgTe [4] , [5] . Common to all these materials is the presence of heavy elements with a reasonably large atomic spin–orbit interaction (SOI). Such a similarity arises from the fact that in all TI systems, the bulk band gap is the result of band inversion by SOI [4] . In other words, without such a SOI-induced band inversion, no topological phase can be realized in a system. In a more general context, SOI tends to lift the degeneracy of energy bands. In systems with inversion ( I ) symmetry, such a splitting leaves the energy states spin-degenerate, as long as the time-reversal ( T ) symmetry is hold. T -symmetry connects the states ψ k ,↑ and ψ − k ,↓ , whereas the I -symmetry enforces the degeneracy between ψ k ,↑(↓) and ψ − k ,↑(↓) . Breaking the I -symmetry lifts the latter constraint, and hence, lets the energy bands be spin-split at generic k -points. Rashba spin splitting (RSS) [15] well exemplifies this situation, as described by H R = p 2 /2 m +ν [e ·( s × p )], where e is the direction of the potential gradient, breaking I -symmetry, and s and p are the spin and momentum operators, respectively. This interaction leads to several unique phenomena, such as the spin Hall effect [16] , the spin Galvanic effect [17] and the magneto-electric effect [18] . Furthermore, once superconductivity occurs in a Rashba system, unusual features such as the mixing of the singlet and triplet pair states, a large upper critical field beyond the Pauli limit [19] , [20] and topological superconductivity with the Majorana edge channels [21] can appear. As SOI is responsible for both RSS and non-trivial topology of electronic states in semiconductors, it is therefore of fundamental interest to know how they interplay with each other once they coexist in a system, and more importantly, what the impact of such an interplay is on the electronic structure of bulk and boundary states. The purpose of this work is to study such an interplay in a layered polar compound, BiTeI. Backed by our earlier band structure calculations [22] , [23] , the angle-resolved photoemission spectroscopy measurements [22] , [24] have revealed that the bulk conduction and valence states in BiTeI are subject to a giant RSS of the order of several hundred meV, lying among the highest reported so far. In this work we show, using the first-principles calculations, that by applying a reasonable hydrostatic pressure, P , the material turns into a TI with many interesting features, such as a nearly double enhancement in RSS accompanied with an unconventional metallic behaviour at the quantum phase transition. It is also demonstrated that unlike the I -symmetric TIs, the gapless Dirac states in the TI phase of BiTeI have completely different shapes at different sides of the material. Consequently, here the surface states on both sides can interestingly have the same spin helicity in a rather broad range of energies inside the bulk band gap, in sharp contrast with the centrosymmetric TIs. Basic properties BiTeI belongs to the trigonal space group of P 3 m 1. As shown in Fig. 1a and b , the crystal structure of BiTeI has a non-centrosymmetric layered structure along its crystallographic c axis with three atoms in one unit cell. Within each unit, a Bi atom is sandwiched between one Te and one I, forming a triple layer. Due to the strong covalency and ionicity of Bi–Te and Bi–I bonds, respectively, the bulk crystal intrinsically possesses a polar axis along the z direction. Despite the strong chemical bonding within each triple layer, the adjacent triple layers are weakly coupled via the Van der Waals interaction. From our previous calculations [23] , we know that around the Fermi level E F , all the bands are essentially p -type, with conduction bands dominated by Bi-6 p and valence bands composed of Te-5 p and I-5 p states. Moreover, due to the negative crystal-field splitting (CFS) of the valence bands and positive CFS of conduction bands near E F , in the absence of SOI, the top valence bands (TVBs) and the bottom conduction bands (BCBs) both become p z type (to avoid any confusion they are referred to as p z A and p z B , respectively). These features make the electronic structure of BiTeI similar to that of the well-known TI systems Bi 2 Te 3 and Bi 2 Se 3 (ref. 6 ). However, here, because of the absence of I -symmetry, it is not possible to assign a distinct even or odd parity to each band. It is also worth noting that in the case of BiTeI, the minimum energy gap E G is not at the Brillouin zone (BZ) centre Γ, but near the hexagonal face centre of the BZ, A point, where k x = k y =0 and k z =π/ c , as shown in Fig. 1c . As will be shown below, because of the latter difference, BiTeI in TI phase shows a rather different topological order from what has been found for Bi 2 Te 3 and Bi 2 Se 3 . Introducing SOI, both spin and orbital mixings are allowed. Consequently, p z A ( p z B ) transforms to thereby getting energetically repelled upward (downward). This accordingly closes the band gap from 1.2 eV down to 0.286 eV and induces a giant bulk RSS among these two sets of bands around point A (ref. 23 ). Despite such a huge reduction in E G , BiTeI remains a trivial insulator as E G still originates from the atomic orbital hybridization between Bi and its neighbouring Te and I atoms. The respective band diagram is shown in Fig. 1d . 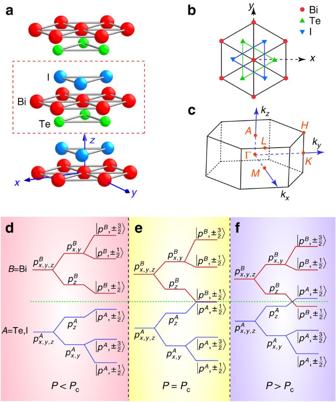Figure 1: Crystal structure, BZ and schematic diagram of band splitting. (a) Crystal structure of BiTeI. A triple layer with Te-Bi-I is indicated by the purple square. (b) The relative in-plane positions of Bi, Te and I as seen along thezaxis. (c) The corresponding BZ. The pressure-induced evolution of BiTeI from a trivial insulator to a TI is schematically drawn in (d–f). In each panel, the evolution of atomic p orbitals into the conduction and valence bands of BiTeI is described as the CFS and spin–orbit coupling are turned on in sequence. As shown in (d) belowPc, the bulk band gapEGis trivial due to the chemical bonding. AtPc, as depicted in (e), a gapless state is realized. Eventually, for pressures beyondPc, the band diagram in (f) shows a band inversion aroundEF, characterizing a topological insulating phase in BiTeI. Here, ±1/2 and ±3/2 indicate thezcomponent of the total angular momentum. Figure 1: Crystal structure, BZ and schematic diagram of band splitting. ( a ) Crystal structure of BiTeI. A triple layer with Te-Bi-I is indicated by the purple square. ( b ) The relative in-plane positions of Bi, Te and I as seen along the z axis. ( c ) The corresponding BZ. The pressure-induced evolution of BiTeI from a trivial insulator to a TI is schematically drawn in ( d – f ). In each panel, the evolution of atomic p orbitals into the conduction and valence bands of BiTeI is described as the CFS and spin–orbit coupling are turned on in sequence. As shown in ( d ) below P c , the bulk band gap E G is trivial due to the chemical bonding. At P c , as depicted in ( e ), a gapless state is realized. Eventually, for pressures beyond P c , the band diagram in ( f ) shows a band inversion around E F , characterizing a topological insulating phase in BiTeI. Here, ±1/2 and ±3/2 indicate the z component of the total angular momentum. Full size image Topological phase transition in BiTeI under pressure Our strategy to turn BiTeI into a TI is to modify its chemical bonds by applying an external hydrostatic pressure. As schematically shown in Figure 1d–f , through this modification, we can effectively control both CFS and SOI such that at a critical pressure P c , become degenerate, whereas at higher P 's their energy ordering is reversed, thereby forming an inverted band gap. Controlling CFS by P is rather easy to understand, because any change in the Bi–Te and Bi–I bonds leads to a change in the energy splitting of and states. For example, our non-relativistic band structure calculations reveal that at P c , the CFS of TVBs is so enhanced that, E G is reduced by 200 meV (see the Supplementary Fig. S1 ). Any band-gap narrowing associated with the CFS modification can be further enhanced through a subsequent enhancement of RSS of and states. As described in detail in Bahramy et al . [23] , this is due to the fact that these two states are symmetrically of the same character, and hence, can very effectively couple with each other through a Rashba-type Hamiltonian if they are energetically close to each other. In other words, the closer they are to each other, the larger RSS would be achieved. To elucidate this mechanism, we show in Fig. 2a–c the respective electronic band dispersions of TVBs and BCBs along the high-symmetry direction H – A – L of BiTeI as hydrostatically compressed by V / V 0 =1, V / V 0 =0.89 and V / V 0 =0.86, where V 0 corresponds to the lattice volume at ambient pressure, P ambient . As shown, at P ambient ( V / V 0 =1), a comparable giant RSS can be seen for both sets of bands with an E G of 286 meV. The corresponding Rashba energy E R , defined as the energy difference between the conduction band minimum (CBM) and the conduction band crossing point, is nearly 110 meV, in perfect agreement with that observed by the angle-resolved photoemission spectroscopy measurements [22] . Compressing the volume down to V / V 0 =0.89, E R monotonically increases until it reaches 200 meV, astonishingly about two times larger than that at P ambient , as shown in Fig. 2b (for a detailed comparison, see Supplementary Fig. S2 also). At this point, the system reaches its quantum critical point, represented by a full band gap closing along the A – H directions. It is worth noting that such a quantum phase transition in BiTeI differs from that in usual centrosymmetic TIs, as there, it is mediated through a band gap closing at a single high-symmetry k -point, for example, the Γ point [25] , [26] , whereas in BiTeI, as will be shown shortly, due to the spin splitting, the band gap is closed at six k -points, all along A – H directions. Thus, they are describable by six 2×2 Dirac Hamiltonians. Here it is important to stress that because of the T -symmetry, these six k -points are two-by-two paired with each other; therefore, their corresponding states form three pairs of 2×2 Dirac fermions. As the band touching is mediated through odd number of such pairs, the transition to TI phase is in principle allowed. Further increasing P , E R starts decreasing and an inverted band gap emerges between the TVBs and BCBs. 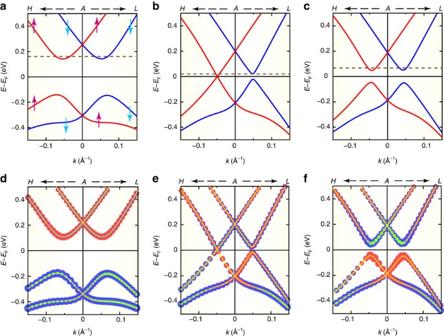Figure 2: Effect of pressure on the bulk electronic states. Electronic dispersions of the Rashba-split BCBs and TVBs in BiTeI as hydrostatically compressed by (a)V/V0=1, (b)V/V0=0.89 and (c)V/V0=0.86. As shown atV/V0=0.89, a band touching between BCBs and TVBs occurs along theH–Adirection. The dashed (brown) line indicates the position of a chemical potential 20 meV above the corresponding CBM of each case. In (a), the spin directions are defined such that they are perpendicular to thekzaxis, as well as their correspondingk-vector. The orbital characteristics of BCBs and TVBs of (a), (b) and (c) are shown in (d), (e) and (f), respectively. The red, blue and green balls correspond to Bi-6p, Te-5pand I-5pstates, respectively. Figure 2d–f demonstrates the orbital characteristics of BCBs and TVBs at V / V 0 =1, V / V 0 =0.89 and V / V 0 =0.86, respectively. A thorough analysis of these bands reveals a clear change in their atomic orbital characteristics as a function of V / V 0 . Although at V / V 0 =1, the BCBs and TVBs are dominated by Bi-6 p and Te-5 p , respectively, at V / V 0 =0.89, they appear to share rather the same orbital characters near the band touching point. On the other hand, at V / V 0 =0.86, one can clearly see that Bi-6 p orbitals now contribute more significantly to TVBs, whereas the BCBs become strongly dominated by Te-5 p and I-5 p states, a clear indication that a band inversion has happened, and hence, the system is now in the TI phase. It is worth adding that in other parts of BZ, including the plane encompassing Γ, M and K , the band gap remains finite for the whole range of P 's. Figure 2: Effect of pressure on the bulk electronic states. Electronic dispersions of the Rashba-split BCBs and TVBs in BiTeI as hydrostatically compressed by ( a ) V / V 0 =1, ( b ) V / V 0 =0.89 and ( c ) V / V 0 =0.86. As shown at V / V 0 =0.89, a band touching between BCBs and TVBs occurs along the H – A direction. The dashed (brown) line indicates the position of a chemical potential 20 meV above the corresponding CBM of each case. In ( a ), the spin directions are defined such that they are perpendicular to the k z axis, as well as their corresponding k -vector. The orbital characteristics of BCBs and TVBs of ( a ), ( b ) and ( c ) are shown in ( d ), ( e ) and ( f ), respectively. The red, blue and green balls correspond to Bi-6 p , Te-5 p and I-5 p states, respectively. Full size image To make sure that BiTeI for P > P c becomes a TI, we have calculated the so-called topological invariant of the whole system when hydrostatically compressed by V / V 0 =0.86. By definition, for three-dimensional systems, the topological invariant is determined by four indices, among which one is called the strong topological index ν 0 , and the three others are weak topological indices ν 1 , ν 2 and ν 3 [4] . The complete list is then described as = ν 0 ; ( ν 1 ν 2 ν 3 ). For a normal insulator, all the four indices are zero, whereas a strong TI is characterized by ν 0 =1. If ν 0 =0, but any of ν 1–3 is 1, the corresponding system is called a weak TI. For the numerical computation of the invariants, several approaches have been proposed [27] , [28] , [29] , [30] . Here we follow the approach introduced in Soluyanov and Vanderbilt [27] (see the Supplementary Methods and Supplementary Fig. S3 for a full description of our computational method for the calculation of the topological invariants). Our calculations show that at V / V 0 =0.86, BiTeI belongs to =1; (001). This clearly indicates that it is a strong TI. Interestingly, the corresponding ν 3 turns out to be 1, which can be attributed to the band touching in the hexagonal face of BZ with k z =π/ c , encompassing A and H points. The interference between the physics of strong and weak TIs could be therefore an interesting problem here. For example, ν 3 =1 means that the one-dimensional conduction channel can appear by dislocations with a Burger's vector along the z axis [31] . Thus, the present system may offer an ideal medium to study the interaction between the surface Dirac fermion as guaranteed by ν 0 =1 and such a 1D channel. 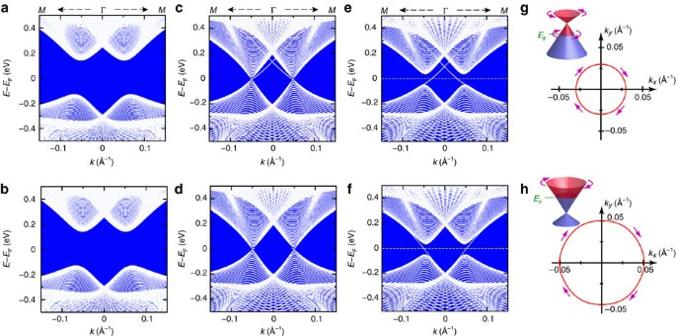Figure 3: Effect of pressure on the surface states. Electronic band dispersions nearEFas obtained for the I-terminated side (top panels) and Te-terminated side (bottom panels) of BiTeI, hydrostatically compressed by (a,b)V/V0=1, (c,d)V/V0=0.89 and (e,f)V/V0=0.86. The Fermi surfaces corresponding to (e) and (f) are shown in (g) and (h), respectively. As depicted schematically in the insets, for an arbitraryEFlocated at the middle of the bulk gap, the Fermi surface at the I-terminated side has a completely different shape from that of the Te-terminated side, but interestingly, for both sides, the same spin helicities are seen. To further confirm that BiTeI becomes a TI for P > P c , we next show in Figure 3 the surface band structures corresponding to the I- and Te-terminated sides of BiTeI. Although the surface states are fully gaped at P ambient , a gapless state appears for both sides at P c . At higher pressures, as shown for the case of V / V 0 =0.86, gapless surface states appear within the bulk band gap. A clear indication that BiTeI has now become a strong TI, thereby further confirming the results of our invariants calculations. Interestingly, the shape of the Dirac surface states at the Te-ended side of BiTeI completely differs from that at the I-ended one. Although for the former, the Dirac point is deeply buried inside the energy valley formed by the Rashba-split TVBs (resembling the Dirac surface states in Bi 2 Te 3 ), on the other side, the Dirac point is energetically well above the bulk CBM. By increasing P , due to the reduction of RSS and the subsequent increase in E G , the latter Dirac point becomes energetically closer to CBM. We expect this to be a characteristic feature for all non-centrosymmetric TI candidates, making them distinguishable from I -symmetric TI systems. As a consequence, in a non-centrosymmetric TI, the electrons are fractionalized into nonequivalent halves on the top and bottom surfaces. This would lead to some novel features and new spintronics functionalities. As shown in Figure 3g and h , the surface Dirac fermions show the similar spin polarization patterns at the top and bottom surfaces, in sharp contrast to the centrosymmetric TIs. It is to be noted that for some thin slabs of Bi 2 Se 3 and Bi 2 Te 3 , such an effect appears to happen when the equivalence of the two surfaces is lifted, for example, by applying an electric field [32] or by differing chemical functionalization [33] . Because of this effect, the Dirac point traverses across the bulk band gap on going from the top side to the bottom side, and always crosses E F on the side surface as long as E F is within the bulk gap. Therefore, if one applies a magnetic field or dopes magnetic impurities, an insulating stripe is expected to appear on the side surface (as E F is now located inside the energy gap of the side surface Dirac fermion). Also, the giant spin Galvanic effect is expected, as the current–spin relation of the top side is same as that of the bottom side. When the hybridization between the Dirac fermions at the top and bottom surfaces occurs, in the momentum space, a gap appears along a one-dimensional (nearly) circular path, resulting in the divergence of the density of states. This accordingly leads to the enhanced electron correlation effect, and consequently, to the excitonic instability. These are just a few examples of the novel phenomena expected in the non-centrosymmetric TIs. Figure 3: Effect of pressure on the surface states. Electronic band dispersions near E F as obtained for the I-terminated side (top panels) and Te-terminated side (bottom panels) of BiTeI, hydrostatically compressed by ( a , b ) V / V 0 =1, ( c , d ) V / V 0 =0.89 and ( e , f ) V / V 0 =0.86. The Fermi surfaces corresponding to ( e ) and ( f ) are shown in ( g ) and ( h ), respectively. As depicted schematically in the insets, for an arbitrary E F located at the middle of the bulk gap, the Fermi surface at the I-terminated side has a completely different shape from that of the Te-terminated side, but interestingly, for both sides, the same spin helicities are seen. Full size image Estimation of P c Let us now briefly discuss on the possible value of P c required for topological phase transition. Performing two sets of volume optimization calculations using the local density approximation (LDA) and generalized gradient approximation (GGA), and then fitting the respective free energies E ( V ) to the Murnaghan equation of state [34] (see Fig. 4 ), we estimate the upper and lower limits of the bulk modulus B 0 of BiTeI to be ~21.9 and ~8.9 Gpa, respectively. The respective LDA and GGA values of the pressure derivative of the bulk modulus B ′ 0 are similarly found to be 7.7 and 7.8, respectively. As mentioned above, our calculations indicate that at P c , V is compressed by 11%. Using the relation [34] P c is accordingly expected to be in the range of 1.7–4.1 GPa. Given that this range of P 's is rather easily affordable in the laboratory, we thus hope this work would stimulate experimentalists in this field to explore such an intriguing topological insulating phase in BiTeI. 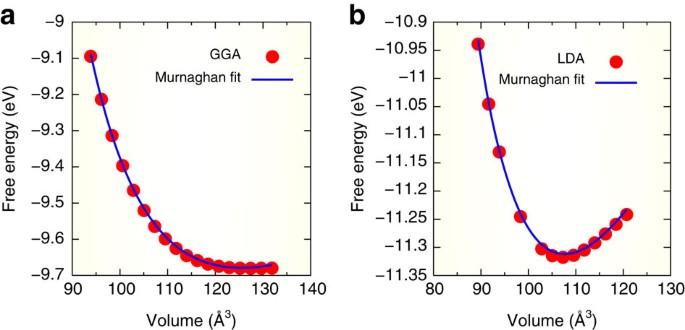Figure 4: Volume dependence of the free energy. Volume dependence of free energyE(V) as obtained from (a) GGA and (b) LDA calculations. To estimate the upper and lower limits of bulk modulusB0and the corresponding pressure derivatives of bulk modulusB′0, the corresponding GGA and LDA data are fitted to the Murnaghan equation of state (solid line). Figure 4: Volume dependence of the free energy. Volume dependence of free energy E ( V ) as obtained from ( a ) GGA and ( b ) LDA calculations. To estimate the upper and lower limits of bulk modulus B 0 and the corresponding pressure derivatives of bulk modulus B ′ 0 , the corresponding GGA and LDA data are fitted to the Murnaghan equation of state (solid line). Full size image At this point, it is worth explaining why BiTeI becomes gapless only at a certain P c , but not for a range of P 's as discussed before [35] , [36] and why such a gapless state occurs along a specific direction. Group theory is the key to answer these questions. Let us first explain the role of crystalline symmetry for the development of dispersion minima (maxima) at BCB (TVB) along particular directions. As already mentioned, BiTeI belongs to C 3 v symmetry consisting of a three-fold rotation C 3 along the z direction and three mirror operations M : y →− y , where y is along the A – H directions. For spin 1/2 electrons, C 3 and M can be represented as and i σ y , respectively, where σ x,y,z are the Pauli matrices for spin degrees of freedom. Additionally, T operator can be defined as i σ y K , where K is the complex conjugation. We can then construct a two band Hamiltonian H c ( k ) for the BCBs invariant under C 3 , M and T . Up to cubic terms of k , it turns out to be: where and are the in-plane and out-of-plane effective masses of the BCBs and ν k,c = ν c (1+α c k 2 ), respectively. Note that in a similar manner, one can construct H v ( k ) for the TVBs. The third term in H c ( k ) is obviously the Rashba term allowing a cylindrical in-plane spin splitting within the k x,y plane. The fourth term, hereafter referred to as H w ( k ), acts as a warping term, trigonally distorting the energy bands. Because of H w ( k ), the inner and outer branches of the Rashba-split conduction bands are distorted in a way that by approaching CBM, they first merge together at the k -points along the A – L directions and then form six energy pockets, each of which is centred along one of the six A – H directions, as shown in Fig. 5a . Exactly at CBM, these six pockets reduce to six points. In the same manner, H w ( k ) distorts TVBs such that the valence band maximum appears as a point similarly lying along A – H . This accordingly explains why band touching between TVBs and BCBs occurs along the A – H direction at P c . It is to be noted that as a direct result of H w ( k ), the energy gap along the A – L directions is always larger than that along the A – H directions for the whole range of P 's, as shown in Fig. 2 and also in the Supplementary Fig. S2(e) . Accordingly, neither at P c nor at any other P the band touching can happen along the A – L directions. The effect of P is to enhance λ for P ≤ P c , such that at the band-touching points, one can clearly see a rather large gap (as large as 40 meV) along the A – L directions where the H w contribution is zero. 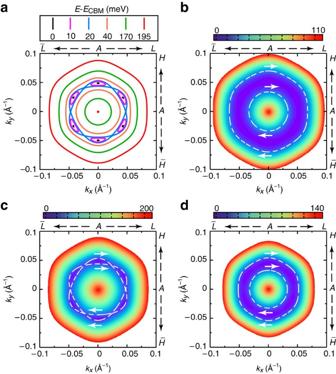Figure 5: Energy evolution of the conduction bands. (a) Energy isocontours corresponding to various chemical potentials above CBM of BiTeI, withV/V0=0.89. In (b), (c) and (d), the respective energy spectra of BCBs mapped into theAplane (kx,ky,kz=π/c) of BiTeI withV/V0=1,V/V0=0.89 andV/V0=0.89 are shown. The upper limit of energy (represented by the red colour) corresponds to the Rashba energyERof BCBs at the givenV/V0. The dashed lines indicate the isocontours of energy for a chemical potential fixed at 20 meV above the CBM of each case. Arrows denote the spin directions. Such a warping effect and its enhancement at the quantum critical point can be well understood by comparing Figure 5b–d , in which the isocontours of energy for an arbitrary E F fixed at 20 meV above the CBM (corresponding to the dashed brown lines in Fig. 2 ) are shown at different P 's. As can be seen, at P c , the inner and outer branches of the Rashba-split conduction bands are just about to form the six energy pockets, whereas away from P c , they form two distinct rings among which the outer one appears to be more significantly distorted by H w . Figure 5: Energy evolution of the conduction bands. ( a ) Energy isocontours corresponding to various chemical potentials above CBM of BiTeI, with V / V 0 =0.89. In ( b ), ( c ) and ( d ), the respective energy spectra of BCBs mapped into the A plane ( k x , k y , k z =π/ c ) of BiTeI with V / V 0 =1, V / V 0 =0.89 and V / V 0 =0.89 are shown. The upper limit of energy (represented by the red colour) corresponds to the Rashba energy E R of BCBs at the given V / V 0 . The dashed lines indicate the isocontours of energy for a chemical potential fixed at 20 meV above the CBM of each case. Arrows denote the spin directions. Full size image Let us now address the first question, that is, why the gapless state in BiTeI can be realized only at a certain P c , but not for a range of P s. For the description of gap-closing, we can focus on the two bands touching at P c among the four bands near the chemical potential. Generally, the topological phase transition in time-reversal invariant, non-centrosymmetric systems can be described by using a two-band Hamiltonian where τ 1,2,3 are the Pauli matrices and τ 0 is the unit matrix. The real functions f 0,1,2,3 depend on the three momenta k =( k x , k y , k z ) and P , and are assumed to take into account the interaction of conduction and valence bands. The topological phase transition through an accidental band touching occurs if and only if the three conditions of f 1,2,3 ( k , P )=0 are satisfied simultaneously in the ( k , P ) space. According to the recent work by Murakami, [35] and Murakami and Kuga [36] , the band touching points, in general, form a curve in the ( k , P ) space, because the three conditions f 1,2,3 ( k , P )=0 cannot uniquely specify the four parameters ( k , P ). Therefore, if the system is free of additional constraints other than the time-reversal symmetry, a gapless metallic phase is expected to appear in a finite range of P Є( P c1 , P c2 ) between the two critical pressures P c1 and P c2 . The occurrence of the single P c in BiTeI is traced back to the fact that the band touching occurs along a particular direction in BZ on which the Hamiltonian has an additional symmetry constraint. Along the A – H line, for example, ( k x , k z )=(0, π/ c ), the system is invariant under the combined operation Ω≡ TM of the T and M symmetries. For T = i σ y K and M = i σ y , Ω is given by K , which imposes the following reality conditions: Because of this reality condition, f 2 ( k y , P )=0 at all points along the A – H direction. Therefore, the band touching can be achieved when the two conditions f 1,3 ( k y , P )=0 are satisfied in the ( k y , P ) space. As the number of conditions to be satisfied is the same as the number of parameters, a gapless phase appears only at a single critical point ( k y ,c , P c ). To conclude, using first-principles calculations we have examined the role of spin–orbit interaction in the giant bulk Rashba semiconductor BiTeI and found that under the application of pressure, it leads the system to be an unusual topological insulator. The novel surface states and quantum critical phenomena are intriguing problems for further studies. The effects of the long-range Coulomb interaction and disorder are, for example, the two important issues remaining to be addressed by both the theory and experiment. Volume optimizations To simulate the effect of P , we optimized the structure of BiTeI crystal at various volumes ranging from V / V 0 =1 to V / V 0 =0.84, where V 0 denotes the volume of BiTeI unit cell at P ambient ( a =4.339 ˚ and c =6.854 ˚). For a given volume, both the atomic positions and crystal's shape were allowed to be fully optimized until the magnitude of force on all ions became less than 0.005 eV ˚ −1 . All the structural optimization calculations were performed using both the LDA functional and GGA functional of Perdew-Burke-Ernzerhof (GGA-PBE) as implemented in the VASP programme [37] , [38] . The corresponding BZ was sampled by a 20×20×20 k -mesh. The respective upper and lower limits of bulk modulus B 0 was estimated by fitting the LDA and GGA–PBE-free energies E ( V ) to the Murnaghan equation of state [34] , using equation (1). To relate the volume changes to P , we then used equation (2). Bulk electronic structure calculations Within the same level of the GGA–PBE theory, the electronic structures of the optimized structures were calculated using the augmented plane wave plus atomic orbitals method as implemented in the WIEN2K programme [39] . For this calculations, the muffin tin radii were set to R MT =2.5 bohr for all the atoms and the maximum modulus of the reciprocal vectors K max was chosen such that R MT K max =7.0. Surface electronic structure calculations To calculate the surface band structure, for each V / V 0 , the corresponding augmented plane wave plus atomic orbitals Hamiltonian was first downfolded into an effective low energy 18×18 tight-binding model, using maximally localized Wannier functions [40] , [41] , [42] . We chose p x , p y and p z states as the projection centres on all I, Te and Bi atoms to span the top 12 valence bands and the 6 lowest conduction bands by our 18×18 models. On the basis of these realistic models, we then constructed large tight-binding supercell Hamiltonians composed of 50 units of BiTeI along its hexagonal c axis. The surface states of each side is then computed by diagonalizing the whole Hamiltonian and projecting the corresponding eigenstates onto the maximally localized Wannier functions of the corresponding surface layer. How to cite this article: Bahramy, M. S. et al . Emergence of non-centrosymmetric topological insulating phase in BiTeI under pressure. Nat. Commun. 3:679 doi: 10.1038/ncomms1679 (2012).